Synthesis of higher carboxylic acids from ethers, CO2and H2 Synthesis of higher carboxylic acids using CO 2 and H 2 is of great importance, because CO 2 is an attractive renewable C1 resource and H 2 is a cheap and clean reductant. Herein we report a route to produce higher carboxylic acids via reaction of ethers with CO 2 and H 2 . We show that the reaction can be efficiently catalyzed by an IrI 4 catalyst with LiI as promoter at 170 °C, 5 MPa of CO 2 and 2 MPa of H 2 . The catalytic system applies to various ether substrates. The mechanistic study indicates that the ethers are converted to olefins, which are further transformed into alkyl iodides. The higher carboxylic acids are produced by carbonylation of alkyl iodides with CO generated in situ via RWGS reaction. This report offers an alternative strategy of higher carboxylic acid synthesis and CO 2 transformation. As an attractive C1 resource, CO 2 can be converted to various kinds of value-added products [1] , [2] , [3] , [4] , [5] . Carboxylic acids are an important class of chemicals. Synthesis of carboxylic acids using CO 2 as a C1 synthon is an interesting topic. In the past decades, great advances have been made in synthesis of formic acid via CO 2 hydrogenation [6] , [7] , [8] , [9] , [10] . Synthesis of higher carboxylic acids using CO 2 has also been extensively studied [11] , [12] , [13] , [14] , [15] , [16] , [17] . However, at present stage expensive or air/water sensitive substrates, such as Grignard and other organometallic reagents, unsaturated hydrocarbons and/or organic halides, were usually used in stoichiometric reactions. Moreover, silanes and/or metallic reducing agents were often required to produce higher carboxylic acids. Hydrogen gas is a clean, cheap and easily available reductant. Undoubtedly, synthesis of higher carboxylic acids using CO 2 and H 2 is of great importance. In a pioneering work, higher carboxylic acids were successfully synthesized by reaction of olefins, CO 2 and H 2 using four-component catalytic system, containing {RhCl(CO) 2 } 2 catalyst, PPh 3 ligand, CH 3 I promoter, and acidic additive (p-TsOH·H 2 O) [18] . Later, it was reported that acetic acid (AcOH) could be produced via methanol hydrocarboxylation with CO 2 and H 2 at above 180 °C, which was accelerated by Ru-Rh bimetallic catalyst, imidazole ligand and LiI promoter [19] . This reaction could also be efficiently accelerated by Rh catalyst, in the presence of 4-methylimidazole ligand, LiCl and LiI promoters [20] . Therefore, in the previous reports of higher carboxylic acid synthesis using CO 2 and H 2 , Rh-based four catalytic components were used to accelerate the reaction. Ethers are cheap and basic chemicals that can be obtained from various sources including biomass, but they have not been utilized as substrate in producing higher carboxylic acids with CO 2 . In general, ethers are less reactive than olefins and/or alcohols. Herein we report a strategy to produce higher carboxylic acids from ethers, CO 2 and H 2 . The reaction can be effectively accelerated by a simple catalytic system consisting of IrI 4 catalyst and LiI promoter at 170 °C (Fig. 1 ). The catalytic system has good substrate adaptability and various ethers could be converted to higher carboxylic acids. 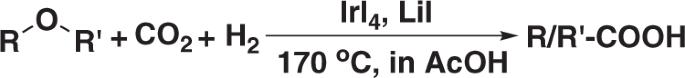Fig. 1 Synthesis of higher carboxylic acids via reaction of ether with CO2and H2. Higher carboxylic acids can be efficiently produced from ether, CO2and H2, where a simple Ir catalyst was utilized. This route is of practical importance because some of the higher carboxylic acids are much more valuable than the corresponding ether substrate (Supplementary Table 1 ). In addition, the price of Ir is much lower than that of Rh although both are known as noble metals. Fig. 1 Synthesis of higher carboxylic acids via reaction of ether with CO 2 and H 2 . Higher carboxylic acids can be efficiently produced from ether, CO 2 and H 2 , where a simple Ir catalyst was utilized. Full size image Catalytic system Tetrahydrofuran (THF) is a bulk chemical, which can be obtained from various feedstocks including biomass [21] . In addition, the C 5 carboxylic acids are much more expensive than THF. Therefore, we adopted THF as model ether to study the catalytic system (Table 1 ). The reaction could be efficiently accelerated by IrI 4 catalyst and LiI promoter in AcOH solvent at 170 °C, and the yield of C 5 carboxylic acids reached 70% after 16 h (entry 1). The products contained two isomers, i.e., pentanoic acid and 2-methylbutanoic acid, and their molar ratio was 58:42. A little C 6 carboxylic acids were also formed in the reaction. The rest of the THF substrate was converted to butane. In addition, trace of methane was also detected. 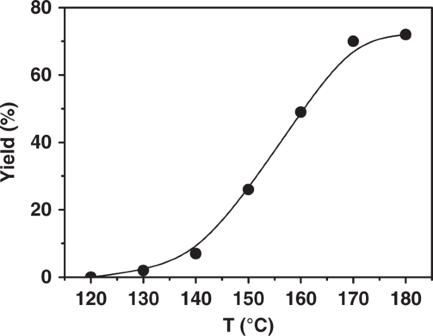Fig. 2 Impact of reaction temperature. Reaction conditions: 20 μmol IrI4, 2 mmol LiI, 0.6 mL AcOH, 2.45 mmol THF, 5 MPa CO2(68 mmol) and 2 MPa H2(at room temperature), 16 h. We also tried different Ir catalyst precursors, such as Ir(CO)(PPh 3 ) 2 Cl, Ir(CO) 2 (acac), and IrCl 3 , the results indicated that they were not as efficient as IrI 4 (Supplementary Table 2 ). We set the reaction time at 8 h and tested other catalytic systems. The IrI 4 catalyst was essential to the reaction because no target product was observed without it (entries 2–3). The Rh catalyst was effective for synthesis of carboxylic acids via olefin and/or alcohol hydrocarboxylation with CO 2 and H 2 [18] , [19] , [20] . Whereas in this work no product was obtained when RhI 3 was used to replace IrI 4 (entry 4). We also tried other metal compounds, such as CoCl 2 , FeI 2 , RuI 3 , PdCl 2 , and PtCl 2 , but the results were poor (entries 5–9). Hence IrI 4 was a suitable catalyst for this reaction. Table 1 Different catalytic systems for synthesizing C 5 carboxylic acids from THF, CO 2 , and H 2 . Full size table The promoter was also crucial to the reaction. Without LiI, the target reaction did not occur (entry 10). When other alkali metal iodides (NaI, KI) were utilized in the reaction, the yields were much lower than that using LiI (entries 2, 11, 12). Moreover, their promoting effects followed the order: LiI > NaI > KI. We also tested alkaline-earth metal iodide (MgI 2 ) or transition metal iodide (ZnI 2 ), but the C 5 carboxylic acids were not observed (entries 13, 14). The superiority of Li + may lie in its stronger Lewis acidity and small size, which could help to activate the substrate [19] , [20] . When LiCl and LiBr were adopted instead of LiI, the products were hardly detectable (entries 15, 16). We further tried iodine (I 2 ) and organic iodide (CH 3 I), but the results were not satisfactory (entries 17, 18). The iodide effects in organic reactions have been summarized elsewhere [22] . The solvent effect was also studied in this work. When the reaction was conducted in hexanoic acid, instead of AcOH, the reaction took place but the yield was not as high as that in AcOH (entries 2, 19). When other common organic solvents such as DMF, toluene and DMSO were used, the reaction did not occur (entries 20–22). The reaction could not proceed in water either (entry 23). We also tried an ionic liquid, i.e., 1-ethyl- 3 -methylimidazolium acetate, whereas no target product was found after the reaction (entry 24). These suggested that the solvent acidity was crucial to the reaction. 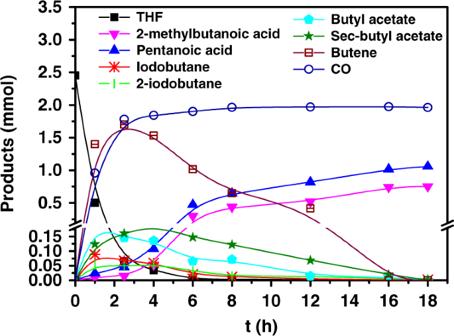Fig. 3 Time course of the reaction. Reaction conditions: 20 μmol IrI4, 2 mmol LiI, 0.6 mL AcOH, 2.45 mmol THF, 5 MPa CO2(68 mmol) and 2 MPa H2(at room temperature), 170 °C. Further experiments indicated that organic acids such as AcOH, CF 3 COOH, or CH 3 SO 3 H could accelerate the reaction and their effects were similar (Supplementary Table 3 ), while the reaction did not take place when an inorganic Bronsted acid (H 3 PO 4 ) or a Lewis acid (Al(OTf) 3 ) was used. This resulted mainly from the better solubility of the reactive components in organic acids. As a cheap, safer and easily available organic acid, acetic acid was the suitable choice of the reaction solvent. In brief, the catalytic system consisting of IrI 4 , LiI, and AcOH was suitable for the reaction. Impact of reaction conditions Based on the above catalytic system, we studied the impact of reaction temperature (Fig. 2 ). The C 5 carboxylic acids appeared at 130 °C, and the yield rose quickly with elevating temperature. At 170 °C, the yield of C 5 carboxylic acids reached 70% and the increase became minor when the temperature was further raised. Consequently, the suitable reaction temperature was 170 °C. At this temperature, we investigated the effect of other reaction conditions, such as dosages of IrI 4 and LiI, pressures of CO 2 and H 2 . 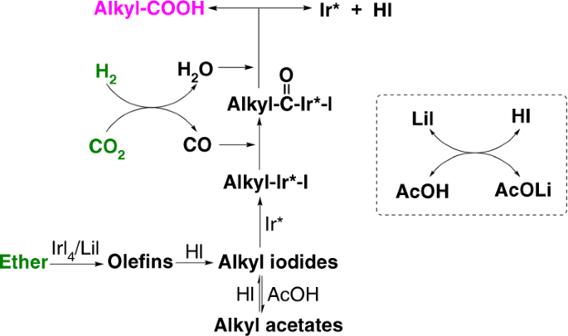Fig. 4 The proposed reaction mechanism. Ir* represents the active center of the Ir catalyst. The ether is converted to olefins, which are further transformed into alkyl iodides. The higher carboxylic acids are produced by carbonylation of alkyl iodides with CO generated in situ via RWGS reaction. The results are shown in Supplementary Table 4 . The yield of C 5 carboxylic acids increased with the elevating IrI 4 dosage, and the yield reached 70% when 20 μmol IrI 4 was used in the reaction (entries 1, 2). Whereas the catalytic performance decreased slightly if the IrI 4 dosage was further raised (entries 3, 4). The dosage of LiI also affected the reaction and the trend was similar to that of IrI 4 (entries 2, 5–7). In addition, the suitable amount of LiI was 2 mmol. The reactant gases were needed in the reaction. Without CO 2 and/or H 2 , no product was observed (entries 8–10). The ratio of CO 2 and H 2 influenced the reaction. We fixed the total pressure at 7 MPa and the best performance was obtained at 5 MPa CO 2 and 2 MPa H 2 (entries 2, 11–13). We further fixed the CO 2 /H 2 ratio at 5/2 and changed the total pressure. It was found that the yield increased with the elevating total pressure, but the increase became minor when the pressure was high enough (entries 2, 14, 15). In short, the optimized reaction condition was 20 μmol IrI 4 , 2 mmol LiI, 0.6 mL AcOH, 2.45 mmol THF, 5 MPa CO 2 (68 mmol) and 2 MPa H 2 (at room temperature), 170 °C. Fig. 2 Impact of reaction temperature. Reaction conditions: 20 μmol IrI 4 , 2 mmol LiI, 0.6 mL AcOH, 2.45 mmol THF, 5 MPa CO 2 (68 mmol) and 2 MPa H 2 (at room temperature), 16 h. Full size image Substrate adaptability Based on above condition, we tested various ether substrates (Table 2 ). The representative GC-MS spectra are given in Supplementary Figs. 1 – 7 . In addition, all the LC-MS graphs of the product were provided in Supplementary Figs. 8 – 33 , the detailed peak information of which was supplied in Supplementary Tables 10 – 35 . When the THF with one or two alkyl substituents were tried, the reaction took place but the yield of products was lower (entries 2, 3). We also tested furan and found that the reaction products and their distribution were similar to those from THF (entries 4). This suggested that furan was in situ reduced to THF before carboxylic acids were formed. After screening the cyclic ethers of different carbon chain length (C 3 , C 4 , C 5 , C 6 ), we observed that they could be effectively transformed into corresponding carboxylic acids with one more C atom (entries 1, 5–7). Interestingly, besides C 4 products, minor C 5 carboxylic acids and trace C 6 carboxylic acids were also formed when 1,3-epoxypropane (C 3 ) was used as substrate (entry 5). Similar phenomena were also observed when other substrates with shorter alkyl chain were utilized. When olefin oxides, i.e., propylene oxide, cyclopentene oxide and cyclohexene oxide, were used as substrate respectively, the reaction proceeded well (entries 8–10). We also tried dioxane and the result showed that C 3 and C 4 carboxylic acids were produced (entry 11). Besides these ethers of cyclic structure, various linear alkyl ethers were transformed into corresponding carboxylic acids (entries 12–19). The ethers involved different kinds of alkyl groups, such as linear/branched alkyls, primary/secondary alkyls, and/or cycloalkyl. From these catalytic results, we can deduce that both alkyl groups in each ether participated in forming carboxylic acids. The catalytic system could also apply to various aryl alkyl ethers (entries 20–26). The alkyl group could be transformed into corresponding carboxylic acids, while the aryl group was converted to phenol and/or phenyl acetate. The presence of substituents on the benzene ring affected the yield of the carboxylic acids. The yield of the carboxylic acids slightly increased in the presence of an electron withdrawing group, while it decreased remarkably when an electron-donating group was present. Interestingly, the distribution of the product isomers in all cases of Table 2 was largely independent of the original alkyl structures. Table 2 Synthesis of higher carboxylic acids using various ether substrates. Full size table Reaction mechanism Figure 3 depicts the time course of the reaction. Interestingly, THF was quickly and high selectively converted to butene, including 1-butene, cis-2-butene and trans-2-butene, at the beginning of the reaction (Supplementary Fig. 34 ). The butene was further transformed into butyl/sec-butyl acetates and/or iodobutane/2-iodobutane. After the emergence of the acetates and alkyl iodides, the C 5 carboxylic acids, i.e., pentanoic acid and 2-methylbutanoic acid, were observed and their amount increased rapidly. The amount of butene dropped remarkably with the reaction going on, while the amount of acetates and alkyl iodides kept at a much lower level all the time. These phenomena suggested that THF was converted to C 5 products via butene, butyl/sec-butyl acetates and/or iodides. Besides, CO appeared at the start of the reaction, and reached a stable level quickly. This indicated that CO was also a reactive intermediate. After 16 h, the amount of C 5 carboxylic acids was unchanged because the intermediates derived from THF were nearly completely consumed. Fig. 3 Time course of the reaction. Reaction conditions: 20 μmol IrI 4 , 2 mmol LiI, 0.6 mL AcOH, 2.45 mmol THF, 5 MPa CO 2 (68 mmol) and 2 MPa H 2 (at room temperature), 170 °C. Full size image Transformation of higher ethers to olefins is still a challenge at present stage, which usually requires high temperature (ca. 450–650 °C) or with low yield (below 30%) [23] , [24] . Very interestingly, butene could be generated very efficiently at much lower temperature in our catalytic system. The high-efficiency generation of butene could be ascribed to the synergy of IrI 4 and LiI (Supplementary Fig. 35 ). The control experiment using toluene as solvent suggested that the solvent acidity was not necessary in converting ether to olefins. Enlightened by the fact that butene engendered at the beginning of the reaction, we used cyclohexene as the substrate at similar condition, which is easier to handle. The result showed that cyclohexanecarboxylic acid was produced in high yield (60%). This supported that butene was a reactive intermediate of the reaction using THF as substrate. Figure 3 also suggests that the alkyl iodides and/or acetates were derived from butene. For longer chain olefins, the isomerization of the double bond usually occurred in the reaction, generating isomerized products [25] . This may account for the formation of butyl and sec-butyl intermediates from butene. Similar intermediates were also detected when other ether substrates were tested. The control experiments indicated that alkyl iodides and acetates could readily transform into each other at the reaction condition. To clarify whether the iodides or the acetates actually participated in the C–C bond formation, we conducted systematic control tests. The results confirmed that the iodides were indispensable in forming the C 5 carboxylic acids (Supplementary Table 5 ). The alkyl acetates may act as a pool to store and protect the alkyl part of the ether during the reaction. Because the alkyl iodides were much easier to be reduced to alkanes in the presence of H 2 (Supplementary Table 6 ). This indicates that the mechanism of olefin transformation in this work is different from that accelerated by Rh catalyst [18] . As shown in Fig. 3 , CO was in situ generated in the reaction. The control test without THF affirmed that CO was produced from CO 2 via RWGS reaction (Supplementary Fig. 36 ). Further experiment showed that THF and CO (1 MPa) as reactants could efficiently generate target C 5 carboxylic acids, and the product distribution was close to that using THF, CO 2 , and H 2 (Supplementary Table 7 , entry 1). The control test indicated that THF was also firstly converted to butene and then participated in further transformation. In contrast, the yield of the C 5 carboxylic acids did not increase obviously when H 2 was charged together with CO (entries 1, 3). Hence the major role of H 2 was to produce CO in RWGS step. Although CO was a key reactive intermediate, too much of it would suppress the reaction due to the catalyst poisoning (entries 2–4). The results of 13 CO 2 and H 2 18 O labeling tests demonstrated that the C = O and OH in the COOH group of the target carboxylic acids were from CO 2 and H 2 O respectively (Supplementary Figs. 37 – 39 ). The GC-MS results of D 2 and D 2 O labeling tests suggest that obvious H-D exchange existed during the reaction (Supplementary Figs. 40 and 41 ). The detailed study of such exchange reactions has been reported elsewhere [26] . Based on the above results and discussion, we rendered the possible reaction mechanism (Fig. 4 ). Firstly, ether substrate is quickly and selectively converted to olefin, which is key to success of this route. The olefin is further converted into alkyl iodides and/or acetates, which can readily transform into each other. Alkyl iodides participate in the C–C bond formation step, while the alkyl acetates act as a temporary pool of the alkyl intermediates. Then oxidative addition of the alkyl iodides to Ir catalyst takes place, which is followed by insertion of CO generated via RWGS reaction. Next step is the reductive elimination of Alkyl-C = O (acyl) in the presence of water formed in situ, where the C 1 -elongated carboxylic acids are produced. Alkyl iodides generally undergo oxidative addition much more readily than alkyl chlorides or bromides, which accounts for the better performance of LiI than LiCl or LiBr. The oxidative addition of alkyl iodide, CO insertion, and reductive elimination of acyl are basic steps in organic reactions catalyzed by transition metal catalysts [27] , [28] , [29] , [30] . Although the Ir catalyzed methanol carbonylation that manufactures acetic acid from methanol and CO has been well studied [27] , [28] , our paper is different from that technology not only in reactants and products but also in catalyst system and reaction pathway. When the ethers with shorter alkyl chains were used as substrate, C 1 -elongated olefins were observed at the beginning of the reaction, which accounts for the formation of C 2 -elongated carboxylic acids (Supplementary Fig. 42 ). The control experiments suggest that CO 2 also takes part in producing the C 1 -elongated olefin intermediates. To better understand the reaction mechanism, we studied the structure of the catalyst after the reaction. The FTIR characterization of the liquid sample demonstrates that cis-[Ir(CO) 2 I 4 ] − existed in the reaction solution (Supplementary Fig. 43 ). The HR-ESI(-)-MS spectra reveal that different [Ir(CO) x I y ] − (x = 1–2, y = 2–4) species were observed, which may be caused by fragmentation of cis-[Ir(CO) 2 I 4 ] − at the testing condition (Supplementary Fig. 44 ). Fig. 4 The proposed reaction mechanism. Ir* represents the active center of the Ir catalyst. The ether is converted to olefins, which are further transformed into alkyl iodides. The higher carboxylic acids are produced by carbonylation of alkyl iodides with CO generated in situ via RWGS reaction. Full size image The catalytic behavior and the catalyst structure characterization after the reaction suggested that the catalyst was stable in the reaction, indicating that the catalyst has potential of reuse. The major obstacle for recycling the homogeneous catalyst is separation of catalyst from the reaction product, and the effective method should be developed for practical application. To study whether our catalytic system can be translated into a heterogeneous mode, we conducted experiments using different heterogeneous Ir catalysts (Supplementary Table 8 ). The results indicated that activated carbon supported Ir catalyst (Ir/AC) could accelerate the reaction, but the efficiency was much lower than that of the homogeneous ones. In summary, we have developed a route to synthesize higher carboxylic acids from ethers, CO 2 and H 2 . The reaction can be effectively accelerated by a homogeneous Ir catalyst. The higher carboxylic acids can be produced at above 130 °C and high yields are obtained at optimized conditions. The catalyst has very good substrate adaptability and various kinds of ethers, such as cyclic ethers, n-alkyl ethers, iso-alkyl ethers and aryl alkyl ethers, can be efficiently converted to corresponding higher carboxylic acids. The target products are produced via tandem reactions. The ether substrate is quickly and selectively transformed into olefin, which is key to the success of this strategy. The olefin is further converted into alkyl iodides and/or acetates. The alkyl iodides participate in the C–C bond formation in the presence of CO generated by RWGS reaction, while the alkyl acetates act as a temporary pool of alkyl part of the ether. The C 1 -elongated carboxylic acids are produced by reductive elimination of acyl in the presence of water formed in situ. This route has great potential of application because cheap and easily available feedstocks are utilized with high efficiency. We believe that this work will trigger more research for CO 2 transformation into value-added chemicals. General information All reagents were commercially supplied and used as received. All the reactions were carried out in a 16 mL Teflon-lined stainless steel batch reactor equipped with a magnetic stirrer. The inner diameter of the reactor was 18 mm. The amount of carboxylic acids in the reaction solution were determined by a liquid chromatograph (LC-10AT, SHIMADZU) equipped with a refractive index detector (RID) and a BP-800 H + carbohydrate column (S/N 23757, Benson polymeric) using dioxane or dimethyl sulfoxide (DMSO) as the internal standard. The column temperature was maintained at 323.15 K. The column was eluted with 5 mmol/L H 2 SO 4 solution at a flow rate of 0.5 ml/min or 1.0 ml/min according to the carboxylic acids analyzed. The reactive intermediates (butyl/sec-butyl acetates and iodobutane/2-iodobutane) in the solution were determined using a gas chromatograph (GC, Agilent 7890B) equipped with a flame ionization detector (FID) and an HP-INNOWAX capillary column (length = 30 m, diameter = 0.25 mm, film = 0.25 μm) using dodecane as the internal standard. The reaction products were identified by GC-MS (SHIMADZU GC-MS-QP2010) using Rtx-WAX column (length = 30 m, diameter = 0.32 mm, film = 0.25 μm) as well as comparing the retention time with the respective standard in the LC or GC traces. The gaseous samples after reaction were detected by a GC (Agilent 7890B) equipped with a TCD detector and a packed column (carbon molecular sieve TDX-01, 3 mm in diameter and 1 m in length) using argon as the carrier gas. The olefins in gaseous sample was determined using a gas chromatograph (GC, Agilent 7890B) equipped with a flame ionization detector (FID) and a GS-Gaspro capillary column (length = 30 m, diameter = 0.32 mm). The amount of butene during the reaction was calculated according to conservation of matter. Liquid 13 C NMR spectra were recorded on Bruck Avance III 400 HD NMR spectrometer. NMR chemical shifts δ are given in parts per million (ppm) relative to tetramethylsilane. Infrared Radiation (IR) spectroscopy were recorded on Bruker Tensor-27 FT-IR Spectrometer. High-resolution electrospray ionization mass spectrometry (HR-ESI-MS) were recorded on Thermo-Exactive. The needle voltage was 3.5 kV. Catalytic reaction Before the reaction, the IrI 4 catalyst, the LiI promoter, the THF substrate and the AcOH solvent were added into the reactor. The above components could be substituted by others if needed. The reactor was sealed and 0.5 MPa of CO 2 was utilized to replace the air in the reactor for two times. Then CO 2 and H 2 of specified pressure at ambient temperature were charged into the reactor, respectively. The reactor was placed in a furnace and was heated to constant temperature, where the stirrer rotated at 800 rpm. When the reaction was finished the reactor was put into an ice-water bath. After cooling, the residual gas in the reactor was discharged, during which the gaseous sample was collected in a gas bag. For LC analysis, the liquid mixture was diluted with 10 mL 1/1 AcOH/H 2 O, followed by addition of 10 µL dioxane or DMSO as the internal standard. For GC analysis, the liquid mixture was diluted with 4 mL acetone, followed by addition of 10 µL dodecane as the internal standard. Before LC or GC, an aliquot of the sample was filtered through syringe filters with hydrophilic PTFE membrane, and the filtrate was immediately injected into the chromatograph.